Rationally tuned micropores within enantiopure metal-organic frameworks for highly selective separation of acetylene and ethylene Separation of acetylene and ethylene is an important industrial process because both compounds are essential reagents for a range of chemical products and materials. Current separation approaches include the partial hydrogenation of acetylene into ethylene over a supported Pd catalyst, and the extraction of cracked olefins using an organic solvent; both routes are costly and energy consuming. Adsorption technologies may allow separation, but microporous materials exhibiting highly selective adsorption of C 2 H 2 /C 2 H 4 have not been realized to date. Here, we report the development of tunable microporous enantiopure mixed-metal-organic framework (M′MOF) materials for highly selective separation of C 2 H 2 and C 2 H 4 . The high selectivities achieved suggest the potential application of microporous M′MOFs for practical adsorption-based separation of C 2 H 2 /C 2 H 4 . Precise control of pore sizes and pore surfaces within porous materials is very important for their highly selective recognition and thus separation of small molecules, but is very challenging and difficult to achieve in traditional zeolite materials [1] . The situation has been changing since the emergence of a new type of porous material, so-called microporous metal-organic frameworks (MOFs) or porous coordination polymers. The pores within porous MOFs, particularly those within isoreticular MOFs whose structures are pre-determined by the coordination geometries of the secondary building blocks, can be systematically modified by changing the organic bridging linkers and controlling the framework interpenetration [2] , [3] , [4] , [5] . Furthermore, the pore surfaces of porous MOFs can be functionalized by the immobilization of different recognition sites, such as open metal sites, Lewis basic/acidic sites and chiral pockets, to direct the recognition of small molecules [6] , [7] , [8] , [9] , [10] , [11] , [12] , [13] , [14] . Systematically tuning micropores can achieve size-specific encapsulation of small gas molecules, and immobilization of functional sites enables varying substrate interactions: microporous MOF materials have emerged as promising microporous media for the recognition and separation of small molecules [15] , [16] , [17] , [18] , [19] , [20] , [21] , [22] , [23] , [24] , [25] , [26] , [27] , [28] , [29] , [30] , [31] , [32] . Kitagawa pioneered the research on construction of porous mixed-metal-organic frameworks (M′MOFs) by making use of M-Salen metalloligands in 2004 (refs 15 , 16 ). Such a novel approach eventually led to few porous M′MOFs for heterogeneous asymmetric catalysis and enantioselective separation [4] , [17] , [18] . Recently, we have successfully developed this metalloligand or pre-constructed building block approach to construct porous MOFs, and realized the first such mixed-metal-organic framework (M′MOF) Zn 3 (BDC) 3 [Cu(SalPyen)]·(G) x (M′MOF- 1 ; BDC=1,4-benzenedicarboxylate; G=guest molecules) with permanent porosity as clearly established by both gas and vapour sorption [32] . This new M′MOF approach has provided us with a new ability to tune and functionalize the micropores within this series of isoreticular M′MOFs by: the incorporation of different secondary organic linkers; the immobilization of different metal sites other than Cu 2+ ; the introduction of chiral pockets/environments through the usage of chiral diamines; and derivatives of the precursor by the usage of other organic groups such as t -butyl instead of methyl group. And thus to explore novel functional microporous M′MOFs for their recognition and separation of small molecules. We initiated studies on such endeavour by making use of Cu-Salen pre-constructed building blocks because of the straightforward and easy synthesis of the Cu-Salen precursors and the resulting porous M′MOFs. To make use of chiral ( R , R )-1,2-cyclohexanediamine to construct the chiral metalloligand Cu(SalPyCy), enantiopure M′MOF Zn 3 (BDC) 3 [Cu(SalPycy)]·(G) x (M′MOF- 2 ), which is isostructural to the nonchiral Zn 3 (BDC) 3 [Cu(SalPyen)]·(G) x (M′MOF- 1 ), can be readily assembled by the solvothermal reaction of this chiral building block with Zn(NO 3 ) 2 and H 2 BDC, leading to the chiral cavities within M′MOF- 2 ( Fig. 1 ). Furthermore, such chiral cavities can be straightforwardly tuned by the incorporation of different bicarboxylate CDC (CDC=1,4-cyclohexanedicarboxylate) for their enhanced recognition and separation of small molecules. 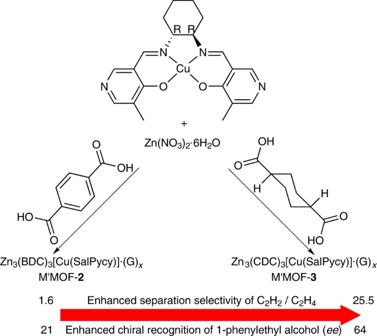Figure 1 Syntheses and separation capacities of M′MOFs-2 and -3. Figure 1 Syntheses and separation capacities of M′MOFs-2 and -3. Full size image Herein, we report the synthesis, structures, sorption and chiral recognition studies on these two new M′MOFs Zn 3 (BDC) 3 [Cu(SalPycy)]·(G) x (M′MOF- 2 ) and Zn 3 (CDC) 3 [Cu(SalPycy)]·(G) x (M′MOF- 3 ). M′MOF- 3 exhibits significantly enhanced selective separation of C 2 H 2 /C 2 H 4 and enatioselective recognition of 1-phenylethyl alcohol (PEA) than M′MOF- 2 , highlighting the first example of microporous materials for highly selective separation of C 2 H 2 /C 2 H 4 , a very important industrial separation. Syntheses and structural characterization of M′MOFs The new Salen-type chiral Schiff base of pyridine derivative H 2 SalPyCy was prepared by condensation of 5-methyl-4-oxo-1,4-dihydro-pyridine-3-carbaldehyde with (1R,2R)-cyclohexanediamine. Reaction of Cu(NO 3 ) 2 ·2.5H 2 O with H 2 SalPyCy formed the pre-constructed building block Cu(H 2 SalPyCy)(NO 3 ) 2 that was easily incorporated into M′MOF- 2 and - 3 by the solvothermal reactions with Zn(NO 3 ) 2 ·6H 2 O and H 2 BDC or H 2 CDC, respectively, in dimethylformamide (DMF) at 373 K as dark-blue thin plates. They were formulated as Zn 3 (BDC) 3 [Cu(SalPyCy)]·5DMF·4H 2 O (M′MOF- 2 ) and Zn 3 (CDC) 3 [Cu(SalPyCy)]·5DMF·4H 2 O (M′MOF- 3 ) by elemental microanalysis and single-crystal X-ray diffraction (XRD) studies, and the phase purity of the bulk material was independently confirmed by powder XRD. The desolvated MMOFs- 2a and - 3a for the adsorption studies was prepared from the methanol-exchanged samples followed by the activation under ultra-high vacuum at room temperature. The XRD profiles of desolvated MMOFs- 2a and - 3a indicate that they maintain the crystalline framework structures ( Supplementary Figs S14–S16 ). X-ray single-crystal structures reveal that M′MOF- 2 and - 3 are isostructural three-dimensional frameworks, in which Zn 3 (COO) 6 secondary building blocks are bridged by BDC or CDC anions to form the 3 6 two-dimensional tessellated Zn 3 (BDC) 3 or Zn 3 (CDC) 3 sheets that are further pillared by the Cu(SalPyCy) ( Fig. 2 , Supplementary Figs S1 and S2 ). Topologically, M′MOF- 2 and - 3 can be described as a hexagonal primitive networks (Schäfli symbol 3 6 4 18 5 3 6), which are the same as its achiral analogue Zn 3 (BDC) 3 [Cu(SalPyen)] (ref. 33 ); however, the incorporation of chiral metalloligand Cu(SalPycy) leads to enantiopure M′MOF- 2 and - 3 , exhibiting two chiral pore cavities of about 6.4 Å in diameter ( Fig. 2a,b ). The chiral pore cavities are filled with the disordered solvent molecules in which M′MOF- 2 and - 3 have the pore accessible volume of 51.7 and 48.1%, respectively, calculated using the PLATON program [34] . 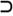Figure 2: X-ray crystal structures of M′MOF-3 and M′MOF-3S-PEA. (a) The hexagonal primitive network topology (Schäfli symbol 36418536) and (b) the three-dimensional (3D) pillared framework with chiral pore cavities for M′MOF-3. (c) The hexagonal primitive network topology and (d) the 3D pillared framework exclusively encapsulating S-PEA molecules for M′MOF-3S-PEA. (Zn, pink; Cu, cyan; O, red; C, grey; N, blue; H, white). Figure 2: X-ray crystal structures of M′MOF-3 and M′MOF-3 S-PEA. ( a ) The hexagonal primitive network topology (Schäfli symbol 3 6 4 18 5 3 6) and ( b ) the three-dimensional (3D) pillared framework with chiral pore cavities for M′MOF- 3 . ( c ) The hexagonal primitive network topology and ( d ) the 3D pillared framework exclusively encapsulating S-PEA molecules for M′MOF- 3 S-PEA. (Zn, pink; Cu, cyan; O, red; C, grey; N, blue; H, white). Full size image Microporous nature of M′MOFs To establish the permanent porosity, the methanol-exchanged M′MOFs- 2 and - 3 were activated under high vacuum at room temperature overnight to form the desolvated M′MOF- 2a and - 3a . Nitrogen adsorption on the activated M′MOFs- 2a and - 3a at 77.3 K was very slow because of the activated diffusion effects. Therefore, CO 2 adsorption at 195 K was used for their pore characterization. Surprisingly, they exhibit remarkably different sorption isotherms attributed to the different dicarboxylates. The uptake of M′MOF- 2a (158 cm 3 g −1 ) is about twice than that of M′MOF- 3a (86 cm 3 g −1 ) at P/P 0 of 1 ( Fig. 3 ). Both M′MOF- 2a and - 3a show hysteretic sorption behaviours, indicating their framework flexibility and the existence of the meta-stable intermediate frameworks, which have been also observed in other flexible porous MOFs [5] . The Langmuir (BET) surface areas calculated from the first step adsorption isotherms are 598(388) and 237(110) m 2 g −1 for M′MOF- 2a and - 3a , respectively, within the pressure range of 0.05< P / P 0 <0.3 ( Supplementary Figs S3–S5 ). Assuming that the second step isotherms still fit into the monolayer coverage model, the overall Langmuir surface areas of M′MOF- 2a and - 3a are 939 and 551 m 2 g −1 . Their total pore volumes from the highest P / P 0 values and pore volumes corresponding to the intermediate isotherm step are 0.301 (0.189) and 0.164 (0.049) cm 3 g −1 for M′MOF- 2a and M′MOF - 3a , respectively. 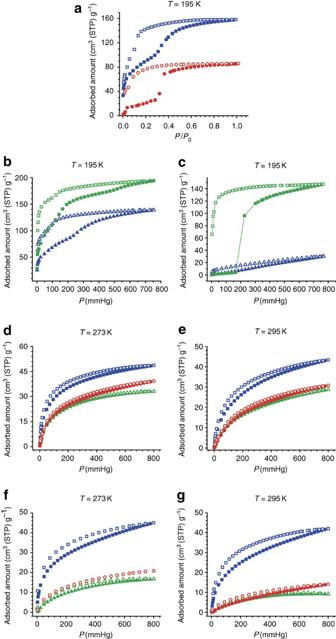Figure 3: Gas sorption isotherms on the two activated M′MOFs at different temperatures. (a) CO2sorption on M′MOFs-2a(blue square) and -3a(red dot) at 195 K. (b) C2H2(green square) and C2H4(blue triangle) on M′MOF-2aat 195 K. (c) C2H2(green square) and C2H4(blue triangle) on M′MOF-3aat 195 K. (d) C2H2(blue square), CO2(red dot) and C2H4(green triangle) on M′MOF-2aat 273 K. (e) C2H2(blue square), CO2(red dot) and C2H4(green triangle) on M′MOF-2aat 295 K. (f) C2H2(blue square), CO2(red dot) and C2H4(green triangle) on M′MOF-3aat 273 K. (g) C2H2(blue square), CO2(red dot) and C2H4(green triangle) on M′MOF-3aat 295 K. Adsorption and desorption branches are shown with closed and open symbols, respectively. Figure 3: Gas sorption isotherms on the two activated M′MOFs at different temperatures. ( a ) CO 2 sorption on M′MOFs- 2a (blue square) and - 3a (red dot) at 195 K. ( b ) C 2 H 2 (green square) and C 2 H 4 (blue triangle) on M′MOF- 2a at 195 K. ( c ) C 2 H 2 (green square) and C 2 H 4 (blue triangle) on M′MOF- 3a at 195 K. ( d ) C 2 H 2 (blue square), CO 2 (red dot) and C 2 H 4 (green triangle) on M′MOF- 2a at 273 K. ( e ) C 2 H 2 (blue square), CO 2 (red dot) and C 2 H 4 (green triangle) on M′MOF- 2a at 295 K. ( f ) C 2 H 2 (blue square), CO 2 (red dot) and C 2 H 4 (green triangle) on M′MOF- 3a at 273 K. ( g ) C 2 H 2 (blue square), CO 2 (red dot) and C 2 H 4 (green triangle) on M′MOF- 3a at 295 K. Adsorption and desorption branches are shown with closed and open symbols, respectively. Full size image Separation of acetylene and ethylene within M′MOFs The unique CO 2 sorption isotherms encouraged us to examine the capacities of M′MOF- 2a and - 3a for their selective separation of C 2 H 2 /C 2 H 4 at 195 K, given the fact that these two molecules have comparable molecular sizes with CO 2 . For M′MOF- 2a ( Fig. 3b ), the shapes of the isotherms are complex, which are apparently attributed to the framework flexibility during adsorption. The total pore volumes were calculated from the highest P / P 0 values ( P / P 0 ∼ 0.99) using densities of 0.577, 0.726 and 1.032 g cm −3 for the densities of C 2 H 4 , C 2 H 2 and CO 2 , respectively. The total pore volumes were 0.306, 0.309 and 0.301 cm 3 g −1 for C 2 H 4 , C 2 H 2 and CO 2 , respectively, which are basically the same, indicating that all three gas molecules can have the full access to the pores within M′MOF- 2a . M′MOF- 3a , however, exhibits significantly different sorption behaviours with respect to C 2 H 4 and C 2 H 2 . M′MOF- 3a can take up the acetylene up to 147 cm 3 g −1 with a one-step hysteresis loop, whereas only small amount of ethylene (30.2 cm 3 g −1 ) without the marked loop at 1 atm and 195 K ( Fig. 3c ). Accordingly, the total pore volumes were different, of 0.066, 0.236 and 0.165 cm 3 g −1 for C 2 H 4 , C 2 H 2 and CO 2 , respectively, as calculated from their highest P / P 0 values, indicating that the three gas molecules have differential degree of access to the pores at 1 atm and 195 K when the pores within M′MOF- 3a become smaller. Such subtle pore control is very important for these kinds of porous materials to exhibit highly selective gas separation. In fact, M′MOF- 2a can only slightly differentiate C 2 H 2 from C 2 H 4 with a low selectivity of 1.6, whereas M′MOF- 3a displays significantly higher selectivity of 25.5 and thus can exclusively separate C 2 H 2 from C 2 H 4 ( Table 1 ). In the diffusion of molecules into spherical or rectangular pores both the cross-section dimensions are important, whereas for slit shaped pores only the smallest dimension is important in determining selectivity. Such significantly enhanced separation capacity of M′MOF- 3a over M′MOF- 2a is attributed to the smaller micropores within M′MOF- 3a , which favours its higher size-specific separation effect on the C 2 H 2 /C 2 H 4 separation. The narrower molecular size of C 2 H 2 (3.32×3.34×5.70 Å 3 ) compared with that of C 2 H 4 (3.28×4.18×4.84 Å 3 ) has enabled the full entrance of the C 2 H 2 into the micropores in M′MOF- 3a , whereas C 2 H 4 molecules are basically blocked or the kinetics are very slow. Table 1 The Henry's constants or the product of the Langmuir equation constants ( q m × b ) and the equilibrium selectivity for gases on the two M′MOFs. Full size table The adsorption isotherms of C 2 H 2 , C 2 H 4 and CO 2 on M′MOF- 2a and - 3a were further measured at 273 and 295 K ( Fig. 3 ). They showed type I sorption isotherms with very little hysteresis. The selectivities towards C 2 H 2 /C 2 H 4 on M′MOF- 2a at 273 and 295 K were 1.5 and 1.9, respectively. Again, M′MOF- 3a exhibited enhanced C 2 H 2 /C 2 H 4 selectivities of 4.1 and 5.2 at 273 and 295 K, respectively; which are 2.5 times higher than the corresponding values for M′MOF- 2a ( Table 1 ). The unique and temperature-dependent gas separation capacities of M′MOF- 3a are attributed both to thermodynamically and kinetically controlled framework flexibility [5] , [26] . The more flexible nature of CDC in M′MOF- 3 has enabled the framework M′MOF- 3 more flexible, thus resulting in narrower pores in activated M′MOF- 3a than those in M′MOF- 2a , as shown in their powder XRD patterns ( Supplementary Fig. S16 ). To open pore entrances for the C 2 H 2 uptake, the gate pressure of 166 mmHg needs to be applied on the thermodynamically flexible framework M′MOF- 3a at 195 K. At higher temperature of 273 and 295 K, the rotation/swing of the organic linker and metalloligand within M′MOF- 3a has enlarged the pore apertures for the access of both C 2 H 2 and C 2 H 4 molecules. Such kinetically controlled framework flexibility has been also revealed in several other porous MOFs and used for their temperature-dependent gas separation [20] , [26] . Interactions of gas molecules with M′MOFs The coverage-dependent adsorption enthalpies of the M′MOFs to acetylene, ethylene and CO 2 were calculated based on the virial method and the van't Hoff isochore. The virial graphs for adsorption of C 2 H 4 , C 2 H 2 and CO 2 on M′MOF -2a and -3a at 273 and 295 K are shown in Supplementary Figures S6–S11 . It is apparent that the virial graphs have very good linearity in the low-pressure region. The parameters and the enthalpies obtained from the virial equation are summarized in Table 2 . For M′MOF- 2a , C 2 H 4 adsorption had A 1 values increasing from −1,770 to −1,551 g mol −1 from 273 to 295 K, which has a similar trend of A 1 values on a carbon molecular sieve increasing from −2,480 to −1,821 g mol −1 from 303 to 343 K (ref. 35 ); C 2 H 2 adsorption had A 1 values increasing from −1,621 to −1,353 g mol −1 from 273 to 295 K, which also has a similar trend of A 1 values on a carbon molecular sieve increasing from −1,444 to −1,302 g mol −1 from 303 to 343 K. It is apparent that the virial parameters for C 2 H 4 and C 2 H 2 adsorption have similar values and trends. CO 2 adsorption on M′MOF- 2a had A 1 values from −1,071 to −940 g mol −1 from 273 to 295 K without well-defined trend, which has been also observed in CO 2 adsorption on a carbon molecular sieve with the A 1 values ranging from −1,000 to −1,045 g mol −1 from 303 to 343 K. The trends in the A 1 parameters for C 2 H 4 , C 2 H 2 and CO 2 adsorption on M′MOF- 2a are consistent with the adsorbate–adsorbate interactions decreasing with increasing temperature. In comparison with those for C 2 H 4 and C 2 H 2 adsorption on M′MOF- 2a , the virial parameters for C 2 H 4 and C 2 H 2 adsorption on M′MOF- 3a are more negative due to its smaller pores, but still have similar values and trends from 273 to 295 K. The fact that the A 1 values for C 2 H 4 adsorption on M′MOF- 3a are not obviously changed indicates that the adsorbate–adsorbate interactions might be independent of temperature from 273 to 295 K ( Supplementary Fig. S11c ). Table 2 Summary of the parameters and the enthalpies of gas adsorption on M'MOFs at 273 and 295 K obtained from the virial equation. Full size table The Q st, n =0 values were 32.7, 37.7 and 32.5 kJ mol −1 for C 2 H 4 , C 2 H 2 and CO 2 adsorption on M′MOF- 2a over the temperature range of 273–295 K. The Q st, n =0 values for C 2 H 2 and CO 2 were comparable to those obtained for their adsorption on a carbon molecular sieve (35.0 kJ mol −1 (C 2 H 2 ) and 28.2 kJ mol −1 (CO 2 )), whereas the value of 32.7 kJ mol −1 for C 2 H 4 adsorption on M′MOF- 2a was significantly lower than the value (50.1 kJ mol −1 ) obtained for C 2 H 4 adsorption on a carbon molecular sieve in the temperature range of 303–343 K. The comparison of the results from the two methods, the linear extrapolation and the virial equation shows that there is a very good agreement ( Fig. 4 ). In all cases the isosteric enthalpies of adsorption gradually decreased with the increasing surface coverage. As expected, the isosteric enthalpies of adsorption are significantly higher than the enthalpies of vaporization of 17, 14 and 16.5 kJ mol −1 for C 2 H 4 , C 2 H 2 and CO 2 , respectively [36] . The isosteric enthalpies of adsorption for C 2 H 2 , C 2 H 4 and CO 2 on M′MOF- 2a are characteristic of their interactions with the hydrophobic pore surfaces presented in carbon molecular sieves. 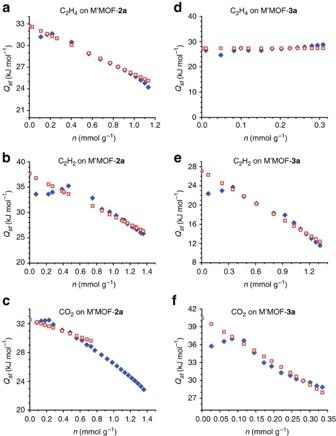Figure 4: Comparison of the gas adsorption enthalpies on the two activated M′MOFs. Ethylene (a,d), acetylene (b,e) and carbon dioxide (c,f) on M′MOF-2a(left) and M′MOF-3a(right) from two methods: the linear extrapolation (blue solid diamond) and virial equation (red open square). Figure 4: Comparison of the gas adsorption enthalpies on the two activated M′MOFs. Ethylene ( a , d ), acetylene ( b , e ) and carbon dioxide ( c , f ) on M′MOF- 2a (left) and M′MOF- 3a (right) from two methods: the linear extrapolation (blue solid diamond) and virial equation (red open square). Full size image The Q st, n =0 for C 2 H 4 , C 2 H 2 and CO 2 adsorption on M′MOF- 3a were 27.4, 27.1 and 40.5 kJ mol −1 , respectively, over the temperature range from 273 to 295 K. The systematically lower Q st, n =0 values for C 2 H 4 and C 2 H 2 adsorption on M′MOF- 3a than those observed on M′MOF- 2a (32.7 kJ mol −1 for C 2 H 4 and 37.7 kJ mol −1 for C 2 H 2 ) may be attributed to the deficiency of π–π interactions between these molecules and CDC moieties on surfaces of pores in M′MOF- 3a . The results derived from the linear extrapolation are in very good agreement with those obtained from the virial equation ( Fig. 4 ). It needs to be mentioned that the Q st values for C 2 H 4 and C 2 H 2 adsorption on M′MOF- 3a are almost the same, indicating that the selective C 2 H 2 /C 2 H 4 separation cannot be realized by their differential interactions with the pore surfaces, thus, the unique gas separation characteristics for M′MOF- 3a are mainly attributed to size-exclusive effect. Enantiopure selective separation of PEA The enantiopure pore environments within M′MOF- 2 and - 3 motivated us to explore their potential for chiral recognition and enantioselective separation. Unlike the achiral M′MOF- 1 Zn 3 (BDC) 3 [Cu(SalPyen)], which encapsulates both R - and S -1-PEA to form Zn 3 (BDC) 3 [Cu(SalPyen)]& R / S -PEA ( Supplementary Fig. S12 ), the enantiopure M′MOF- 3 exclusively takes up S -PEA to form M′MOF- 3 S -PEA (Zn 3 (CDC) 3 [Cu(SalPyCy)]· S -PEA). In fact, the solvothermal reaction of the corresponding reaction mixture of Zn(NO 3 ) 2 ·6H 2 O, H 2 CDC and Cu(H 2 SalCy)(NO 3 ) 2 in the presence of certain amount of racemic PEA in DMF at 100 °C readily formed the enantiopure M′MOF- 3 , which exclusively encapsulates S -PEA ( Fig. 2d ). The incorporated S -PEA can be easily extracted by immersing the as-synthesized M′MOF- 3 S -PEA in methanol. The chiral recognition and enantioselective separation of M′MOF- 2 and - 3 for the R / S -PEA racemic mixture were examined using the bulky as-synthesized materials. The as-synthesized M′MOF- 2 and - 3 were exchanged with methanol and then immersed in the racemic mixture to selectively encapsulate the S -PEA. Once such PEA-included M′MOF- 2 and - 3 were immersed in methanol, the encapsulated PEA within the enantiopure M′MOF- 2 and - 3 can be readily released from the chiral pores, making their potential application for enantioselective separation of R / S -PEA. Chiral HPLC analysis of the desorbed PEA from the PEA-included M′MOF- 2 yielded an ee value of 21.1%, and the absolute S configuration for the excess was confirmed by comparing its optical rotation with that of the standard sample. It must be noted that the used M′MOF- 2 keeps high crystallinity and can be regenerated simply by the immersion into the excess amount of methanol, and thus for further resolution of racemic R / S -PEA. The second and third such regenerated M′MOF- 2 provide an ee value of 15.7 and 13.2%, respectively. The low enantioselectivity of the enantiopure M′MOF- 2 for the separation of R / S -PEA might be attributed to its large chiral pore environments, which have limited its high recognition of S -PEA. The smaller chiral pores within the enantiopure M′MOF- 3 have significantly enhanced its enantioselectivity for the separation of R / S -PEA with the much higher ee value of 64%. The regenerated M′MOF- 3 can also be further used for the separation of R / S -PEA with the slightly lower ee value of 55.3 and 50.6%, respectively. The chiral pores within M′MOF -2 and M′MOF- 3 basically match the size of S -PEA, which are not capable to separate larger alcohol enantiomers, such as 1-(p-tolyl)-ethanol, 2-phenyl-1-propanol and 1-phenyl-2-propanol. Separation of acetylene and ethylene is a very important but challenging industrial separation task. Ethylene, the lightest olefin and the largest volume organic chemical, is largely stocked in petrochemical industry and is widely used to produce polymers and other chemicals [37] . The typical ethylene produced in steam crackers contains on the order of 1% of acetylene [38] , although a p.p.m. level of acetylene (>5 p.p.m.) in ethylene can poison Ziegler-Natta catalyst during ethylene polymerizations and can also lower the product quality of the resulting polymers [39] . Moreover, the acetylenic compounds are often converted into solid, thus blocking the fluid stream and even leading to explosion [40] . There are mainly two commercial approaches to remove acetylenes in ethylene: partial hydrogenation of acetylene into ethylene over a noble metal catalyst such as a supported Pd catalyst [41] , [42] and solvent extraction of cracked olefins using an organic solvent to obtain pure acetylene [43] . However, the former process suffers from the catalyst price and the loss of olefins due to the over hydrogenation to paraffins, although the latter is also disadvantageous in terms of technical and economical aspects, partially, because of the low selectivities of acetylene over olefins and also to the significant loss of solvent after multiple operations. Apparently, there is a significant need to develop novel alternative C 2 H 2 /C 2 H 4 separation approaches. Some recent attempts, hydrogenation by non-precious metal alloy catalysts [44] , ionic liquid extraction [45] , and π-complexation [46] , have been made to reduce the cost or to enhance the selectivities. The realization of our first example of microporous MOF materials for such challenging separation highlights the very promise of the emerging microporous MOFs to resolve this very important industrial separation task in the future. M′MOF- 3a is feasible for C 2 H 2 /C 2 H 4 separation at moderate pressures over 200 mmHg at 195 K. To realize high C 2 H 2 /C 2 H 4 separation at low pressures at 195 K, the gate pressure for the entrance of C 2 H 2 needs to be further reduced, which might be fulfilled by the combinatorial approach outlined in the Introduction. C 2 H 2 /C 2 H 4 separation selectivity of 5.23 has featured M′MOF- 3a as a practical media for this important separation even at room temperature. We have developed the pre-constructed building block approach to introduce chiral pores/pockets within the M′MOFs by the usage of the chiral diamine ( R , R )-1,2-cyclohexanediamine. Such chiral pore/pocket sizes are rationally tuned by the incorporation of different bicarboxylates BDC and CDC within their isostructural M′MOFs Zn 3 (BDC) 3 [Cu(SalPycy)]·(G) x (M′MOF- 2 ) and Zn 3 (CDC) 3 [Cu(SalPycy)]·(G) x (M′MOF- 3 ). The slightly smaller pores within M′MOF- 3 have enabled the activated M′MOF- 3a exhibits much higher separation selectivities with respect to both C 2 H 2 /C 2 H 4 and enantioselective separation of S -1-PEA than M′MOF- 2a , highlighting the very promise of this M′MOF strategy to tune the micropores and immobilize functional sites to direct their specific recognition and thus separation of small molecules. We are now targeting at some more robust porous M′MOFs and immobilizing different metal sites, such as Ni 2+ , Co 2+ , Zn 2+ , Pd 2+ and Pt 2+ , to rationalize the contribution of such open metal sites for their recognition of different small molecules by synthrontron and/or neutron diffraction studies. Furthermore, we will systematically further tune and functionalize the micropores within such microporous M′MOFs by making use of different dicarboxylates such as BDC and CDC derivatives and a variety of metalloligands, and thus to further enhance the C 2 H 2 /C 2 H 4 separation and to target at some other challenging separation tasks, such as O 2 /N 2 , C 2 H 4 /C 2 H 6 and C 3 H 6 /C 3 H 8 separation, and to address some practical enantioselective separation of racemic substrates of industrial and pharmaceutical importance. Materials All reagents and solvents used in synthetic studies were commercially available and used as supplied without further purification. 5-Methyl-4-oxo-1,4-dihydro-pyridine-3-carbaldehyde was synthesized according to the literature procedure [47] . Synthesis of Cu(H 2 SalPyCy)(NO 3 ) 2 A solution of (1R, 2R)-(-)-1,2-cyclohexanediamine (0.846 g, 7.41 mmol) in EtOH (20 ml) was added dropwise to a solution of 5-methyl-4-oxo-1,4-dihydro-pyridine-3-carbaldehyde (1.794 g, 14.82 mmol) in EtOH (130 ml), and the resulting mixture was refluxed for 2 h to form a clear light brown solution. To this solution, a solution of Cu(NO 3 ) 2 ·2.5H 2 O (1.798 g, 7.73 mmol) in EtOH (20 ml) was added, forming a blue precipitate of Cu(H 2 )SalPyCy)(NO 3 ) 2 that was collected by filtration, washed with EtOH and air dried (2.035 g, 51%). Synthesis of Zn 3 (BDC) 3 [Cu(SalPyCy)]·5DMF·4H 2 O A mixture of Zn(NO 3 ) 2 ·6H 2 O (0.236 g, 0.79 mmol), H 2 BDC (0.131 g, 0.79 mmol) and Cu(H 2 SalPyCy)(NO 3 ) 2 (0.143 g, 0.24 mmol) was dissolved in 100 ml DMF, and heated in a vial (400 ml) at 373 K for 24 h. The dark-blue thin plates formed were collected and dried in the air (0.21 g, 57%). Elemental analysis (%): calcd for Zn 3 (BDC) 3 [Cu(SalPyCy)]·5DMF·4H 2 O (C 59 H 77 N 9 O 23 CuZn 3 ): C, 46.02; H, 5.04; N, 8.19; found: C, 45.97; H, 4.98; N, 8.24. Synthesis of Zn 3 (CDC) 3 [Cu(SalPyCy)]·5DMF·4H 2 O A mixture of Zn(NO 3 ) 2 ·6H 2 O (0.236 g, 0.79 mmol), H 2 CDC (0.136 g, 0.79 mmol) and Cu(H 2 SalPyCy)(NO 3 ) 2 (0.143 g, 0.24 mmol) was dissolved in 100 ml DMF, and heated in a vial (400 ml) at 373 K for 24 h. The dark-blue thin plates formed were collected and dried in the air (0.23 g, 62%). Elemental analysis (%): calcd for Zn 3 (CDC) 3 [Cu(SalPyCy)]·5DMF·4H 2 O (C 59 H 95 N 9 O 23 CuZn 3 ): C, 45.48; H, 6.15; N, 8.09; found: C, 45.35; H, 6.23; N, 7.96. Synthesis of Zn 3 (CDC) 3 [Cu(SalPyCy)]· S -PEA·5DMF A mixture of Zn(NO 3 ) 2 ·6H 2 O (0.018 g, 0.06 mmol), H 2 CDC (0.01 g, 0.06 mmol) and Cu(H 2 SalPyCy)(NO 3 ) 2 (0.016 g, 0.30 mmol) was dissolved in 3 ml DMF and 2 ml D,L -PEA, and heated in a vial (23 ml) at 373 K for 24 h. The purple platelet crystals were colleted and dried in the air (0.01 g, 31%). Elemental analysis (%): calcd for Zn 3 (CDC) 3 [Cu(SalPyCy)]· S -PEA·5DMF (C 67 H 97 CuN 9 O 20 Zn 3 ): C, 50.04; H, 6.08; N, 7.84; found: C, 50.12; H, 6.15; N, 7.96. Synthesis of Zn 3 (BDC) 3 [Cu(SalPyen)]· R/S -PEA·5DMF A mixture of Zn(NO 3 ) 2 ·6H 2 O (0.018 g, 0.06 mmol), H 2 BDC (0.01 g, 0.06 mmol) and Cu(H 2 SalPyen) (NO 3 ) 2 (0.015 g, 0.03 mmol) was dissolved in 3 ml DMF and 2 ml D , L -PEA, and heated in a vial (23 ml) at 373 K for 24 h. The purple platelet crystals were colleted and dried in the air (0.01 g, 32%). Elemental analysis (%): calcd for Zn 3 (BDC) 3 [Cu(SalPyen)]· R/S -PEA·5DMF (C 63 H 73 CuN 9 O 20 Zn 3 ): C, 49.26; H, 4.79; N, 8.21; found: C, 49.55; H, 4.85; N, 8.30. Adsorption studies After the bulk of the solvent was decanted, the freshly prepared sample of M′MOF -2 or -3 ( ∼ 0.15 g) was soaked in ∼ 10 ml methanol for 1 h, and then the solvent was decanted. Following the procedure of methanol soaking and decanting for ten times, the solvent-exchange samples were activated by vacuum at room right overnight till the pressure of 5 μmHg. CO 2 , ethylene and acetylene adsorption isotherms were measured on ASAP 2020 for the activated M′MOFs. As the centre-controlled air condition was set up at 22.0 °C, a water bath of 22.0 °C was used for adsorption isotherms at 295.0 K, whereas dry ice-acetone and ice-water bathes were used for the isotherms at 195 and 273 K, respectively. How to cite this article: Xiang, S.-C. et al . Rationally tuned micropores within enantiopure metal-organic frameworks for highly selective separation of acetylene and ethylene. Nat. Commun. 2:204 doi: 10.1038/ncomms1206 (2011).